Observed thinning of Totten Glacier is linked to coastal polynya variability Analysis of ICESat-1 data (2003–2008) shows significant surface lowering of Totten Glacier, the glacier discharging the largest volume of ice in East Antarctica, and less change on nearby Moscow University Glacier. After accounting for firn compaction anomalies, the thinning appears to coincide with fast-flowing ice indicating a dynamical origin. Here, to elucidate these observations, we apply high-resolution ice–ocean modelling. Totten Ice Shelf is simulated to have higher, more variable basal melting rates. We link this variability to the volume of cold water, originating in polynyas upon sea ice formation, reaching the sub-ice-shelf cavity. Hence, we propose that the observed increased thinning of Totten Glacier is due to enhanced basal melting caused by a decrease in cold polynya water reaching its cavity. We support this hypothesis with passive microwave data of polynya extent variability. Considering the widespread changes in sea ice conditions, this mechanism could be contributing extensively to ice-shelf instability. A better understanding of the stability of ice shelves and floating glacier termini is an indispensable element in assessing the mass balance of the Antarctic and Greenland ice sheets and their present and future contributions to sea level change. Increasingly, observational evidence points to enhanced basal melting as a main factor in ice-shelf instability. Such observations include the concurrent thinning of glaciers with floating termini that share the same ocean basins [1] , [2] , [3] , lower thinning rates of adjacent land-terminating glaciers [4] and the retreat of most marine-terminating glaciers along the Antarctic Peninsula [5] . Available oceanographic observations attribute the enhanced melting to either the intrusion of warm waters deep enough to reach the grounding zones or to the modification of surface ocean water properties [6] , [7] , [8] . Totten Glacier (TG) in Wilkes Land discharges the largest volume of ice in East Antarctica at ~70 km 3 y −1 (ref. 9 ). TG forms an ice shelf (TIS) between Law Dome and Sabrina Coast, which is ~2,700 m thick at the grounding line [10] ( Supplementary Fig. S1 ). Moscow University Ice Shelf (MUIS) is located further east on the Sabrina Coast. It has similar areal dimensions to TIS, but a higher thickness at the grounding line (~3,150 m (ref. 10 )). The bedrock beneath large areas of the basins of both glaciers lies below sea level [11] , [12] , which, in the case of increased basal melting, makes their grounding lines susceptible to the hypothesized unstable retreat over inland-deepening bedrock [13] , [14] , [15] , [16] . Such a process would be analogous to the retreat and mass loss of Pine Island Glacier in West Antarctica that have been attributed to the changing geometry of, and enhanced melting in, the sub-ice-shelf cavity [7] . While not much has been reported on the evolution of Moscow University Glacier (MUG), changes near TG over the past decade were noted in large-scale studies of Antarctica. These included net mass loss [9] , [17] , ice surface lowering of the grounded ice [2] , [18] , [19] and thinning of the ice shelf [3] . Our interest in the two glaciers is further motivated by the insights to be gained from comparing their behaviours, given their geographic proximity and the common ocean basin shared by their ice shelves. The outline of this study is as follows. We analyse ICESat-1 laser altimetry observations, corrected by a firn compaction model, to obtain spatial patterns of thickness change. We seek insights into the mechanisms underlying the observed thinning patterns by numerically modelling the ice–ocean interactions with 20 sensitivity experiments using different atmospheric forcings. We assess the simulated melting rates of the two ice shelves by comparing them with rates we independently calculate from ice thickness and InSAR observations of ice velocities. The simulations allow us to identify changes in the volume of cold and saline water produced in polynyas and reaching the sub-ice-shelf cavities as a main factor contributing to the variability of the modelled melting rates. We finally hypothesize on the potential role of this process in the observed thinning, and seek supporting observational evidence from passive microwave data of polynya extents, and from the ICESat-1 measurements of surface elevation changes. Surface elevation change patterns from ICESat-1 We found surface elevation changes from GLAS/ICESat-1 data for the period 2003–2008 and corrected them for decadal firn depth variability ( Fig. 1a,b ). The results have two salient features. The first is a high rate of ice surface lowering in the grounded parts of TG. The other is a marked contrast between this surface lowering and the smaller change observed in the area of MUG. The highest rates of surface lowering in the grounded areas surrounding TG appear to coincide with the fastest flowing ice ( Fig. 1a , inset). Thus, over the 6-year period of the observations, the surface lowered by 80–170 cm y −1 (uncertainty is estimated in the Methods) upstream from the grounding line of the main, fast-flowing trunk of the glacier (location A, Fig. 1a ). Further upstream, and following the curvature of the glacier inland, the surface lowered at a slower rate of 20–50 cm y −1 . Also, upstream from the grounding line of one of the larger, faster-flowing tributary glaciers (location B, Fig. 1a ) the surface lowered by 30–60 cm y −1 over the same period. The robustness of these numbers is supported by the similarity of elevation change rates on either side of the fast-flowing ice areas of between −10 and +20 cm y −1 ( Fig. 1a ). Such low rates of change in the surrounding areas of slow-moving ice mean that variation in local surface mass balance is insufficient to explain the high rates of surface lowering of the fast-flowing ice [4] . This strongly suggests that the observed thinning on the main trunk of the glacier and tributaries is related to ice dynamics. On the floating ice shelf of TG, fewer useful data could be found after applying the signal saturation and cloud filters (see Methods). In addition, the signal of surface elevation is often dominated by the advection of pronounced topographic surface features. We therefore consider only areas where the surface of the ice shelf is relatively smooth as shown by our ICESat-1 surface elevation measurements and satellite imagery ( Fig. 1a ). Accordingly, only a segment directly downstream from the grounding line near location C in Fig. 1a unambiguously exhibits surface lowering of 140–200 cm y −1 . 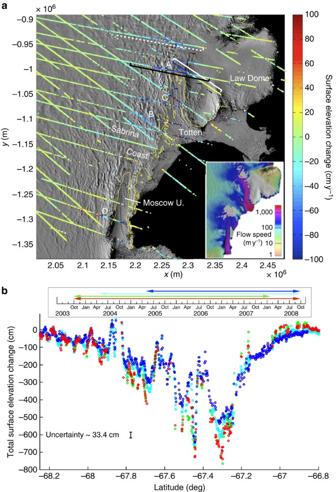Figure 1: Surface elevation changes of Totten and Moscow University glaciers from ICESat-1. Data are from the period 2003–2008 and are corrected for decadal firn depth variability. (a) Changes in surface elevations averaged over the observation intervals. Details of the track combinations used in obtaining surface elevation changes are given inSupplementary Tables S1 and S2andSupplementary Fig. S5. The inset shows the speed field in the area45(grey denotes missing data). White letters mark locations mentioned in the text. The black, white and dotted white lines near location A indicate the sections along which the profiles inFig. 1bandSupplementary Fig. S4are taken. Background image is from MODIS mosaic of Antarctica (MOA)58. Dotted yellow is the grounding line54. (b) Profiles of total surface elevation changes for 4 track combinations (1 (red), 2 (green), 3 (cyan) and 4 (blue);Supplementary Tables S1 and S2) along the section indicated by the black line near location A in (a). The time interval over which surface elevation change was found for each track combination is shown by an arrow with the same color in the box. Figure 1: Surface elevation changes of Totten and Moscow University glaciers from ICESat-1. Data are from the period 2003–2008 and are corrected for decadal firn depth variability. ( a ) Changes in surface elevations averaged over the observation intervals. Details of the track combinations used in obtaining surface elevation changes are given in Supplementary Tables S1 and S2 and Supplementary Fig. S5 . The inset shows the speed field in the area [45] (grey denotes missing data). White letters mark locations mentioned in the text. The black, white and dotted white lines near location A indicate the sections along which the profiles in Fig. 1b and Supplementary Fig. S4 are taken. Background image is from MODIS mosaic of Antarctica (MOA) [58] . Dotted yellow is the grounding line [54] . ( b ) Profiles of total surface elevation changes for 4 track combinations (1 (red), 2 (green), 3 (cyan) and 4 (blue); Supplementary Tables S1 and S2 ) along the section indicated by the black line near location A in ( a ). The time interval over which surface elevation change was found for each track combination is shown by an arrow with the same color in the box. Full size image In the area between the two ice shelves along the Sabrina Coast, lowering rates decrease to ~30 cm y −1 ( Fig. 1a ). Around MUG, most of the grounded ice area exhibits small surface elevation increases of 0–25 cm y −1 . The exception again is the faster-flowing tributary glacier (location D, Fig. 1a ) that is lowering at a rate of ~20 cm y −1 . On the MUIS, the signal is mixed, being affected by surface topography as in TIS, with most points falling between ±50 cm y −1 . The magnitude of the decadal firn depth correction for the ICESat-1 period 2003–2008 is mostly between −30 and +10 cm yr −1 , with the MUG area generally exhibiting larger firn correction values relative to TG owing to larger snowfall variability. The inference that observed thickness is most likely responding to changes in ice dynamics motivates our implementation of ice–ocean modelling, as sustained change in melting and freezing rates at the ice–ocean interface can be a trigger of changes in ice flow. Modelled melting rates at the ice–ocean interface The modelling approach (see Methods) is in effect equivalent to 20 separate simulations of the impact of atmospheric forcing variability on the hydrographic conditions of each year between 1992 and 2011. 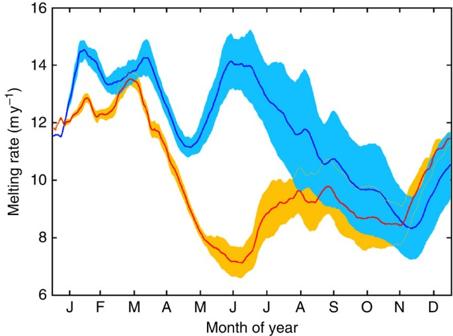Figure 2: Area-averaged melting rates of Totten and Moscow University ice shelves. Averages for each day of the year are calculated over the 20 simulation years 1992–2011 for TIS (blue) and MUIS (red). The coloured areas surrounding the curves represent the s.d. Figure 2 shows the calculated melt rates for both ice shelves, averaged over their respective ice–ocean interface areas. In the following analyses we exclude the results from the first 3 months of each year as they are dominated by the identical initial conditions. The distribution of melting rates in Fig. 2 illustrates two main aspects of the simulation results: the generally higher melting rates of TIS and their larger interannual variability compared with those of MUIS. The difference is most pronounced during the winter months (July, August and September (JAS)). For that period, the simulated TIS melt rates vary between 9.5–15 m y −1 , while those of MUIS are mostly between 7.5–10 m y −1 ( Fig. 2 ). The range of the TIS melt rates appears wider still when including the spring months (October, November and December), with rates between 7 and 11.5 m y −1 , while the corresponding values for MUIS are again mostly between 8 and 10.5 m y −1 ( Fig. 2 ). Figure 2: Area-averaged melting rates of Totten and Moscow University ice shelves. Averages for each day of the year are calculated over the 20 simulation years 1992–2011 for TIS (blue) and MUIS (red). The coloured areas surrounding the curves represent the s.d. Full size image These numbers are reasonably close to the results of our independent calculations from remote-sensing data presented in Table 1 (see Methods). The calculated TIS melting rate of 9.2±0.7 m y −1 falls within the simulated 7–15 m y −1 range. The corresponding observed MUIS melting rate of 5.7±0.6 m y −1 is outside the modelled 7.5–10.5 m y −1 range but near its lower end. Our confidence in the model results is enhanced by the simultaneous agreement of the results for both ice shelves with the independently calculated values given current model limitations, especially the absence of a more reliable bathymetry. Table 1 Average melting rates and the remote-sensing observations used in their calculation. Full size table We seek further insight into the modelling results, in particular the high interannual variability of the TIS melting rates, by comparing the outcomes of two simulations: one with higher average melting rates (year 2009; JAS melting rate=14.7 m y −1 for TIS and 9.8 m y −1 for MUIS), and another with lower average melting (year 2001; JAS melting rate=11.8 m y −1 for TIS and 7.8 m y −1 for MUIS). The spatial distribution of winter melting rates at the ice–ocean interface for both simulation years ( Fig. 3 ) shows that no freezing is simulated underneath either ice shelf. The highest melting rates are located near the eastern margin of both sub-ice-shelf cavities, in the middle and southern sections of TIS, and in the middle section of MUIS ( Fig. 3 ). High basal melting rates in these areas could partially explain the relative smoothness of the corresponding ice-shelf top surfaces in the satellite image ( Fig. 1a ). Higher melting rates in case of TIS, reaching 25 m y −1 in places ( Fig. 3 ), occur at a much larger area of the ice–ocean interface compared with MUIS. In the case of TIS, higher temperatures and higher salinities in the mid-depth parts of the cavity are found in the year 2009 simulation ( Supplementary Fig. S2 ), with winter temperatures between −0.8 and −0.6 °C and a salinity of ~34.5, compared with −1.2 and −0.9 °C and salinity of 34.4 in the year 2001. Spring (figure not shown) exhibits little change in salinity at ~34.4 but a higher temperature again at −1.1 °C in year 2009 compared with −1.4 °C for 2001. In the case of MUIS, temperature and salinity between the 2001 and 2009 simulations change similarly but to a smaller degree. 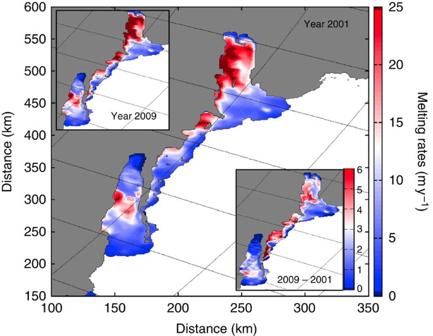Figure 3: Spatial distribution of the simulated melting rates of Totten and Moscow University ice shelves. Melting rates are averaged over July, August and September of each simulation year shown. The main figure is the 2001 simulation, and the top-left inset is the 2009 simulation with the same colour scale as the main figure. The bottom-right inset is the difference in melting rates between the two simulations. Note the different colour scale in the bottom-right inset. Figure 3: Spatial distribution of the simulated melting rates of Totten and Moscow University ice shelves. Melting rates are averaged over July, August and September of each simulation year shown. The main figure is the 2001 simulation, and the top-left inset is the 2009 simulation with the same colour scale as the main figure. The bottom-right inset is the difference in melting rates between the two simulations. Note the different colour scale in the bottom-right inset. Full size image Linking simulated ice-shelf melting and polynya variability The JRA-25 reanalysis data applied as surface forcing produce recurring coastal latent heat polynyas, areas of open water in the sea ice cover, in the vicinity of TIS and MUIS ( Supplementary Fig. S3 ). Sea ice continues to form in these areas of open water but is swept away by offshore winds hence maintaining high rates of air-sea heat and buoyancy loss. As a result of sea ice formation at the surface freezing point accompanied by brine rejection, polynyas become sites of cold, saline water production during winter. The model simulates a more extensive polynya in the year 2001, resulting in colder and more saline water in the polynya area ( Supplementary Fig. S3 ). Temperature–salinity (T–S) diagrams ( Fig. 4 ) elucidate the relationship among polynya water masses, the modified Circumpolar Deep Water (mCDW) prevalent on the continental shelf and the water masses in the TIS sub-ice-shelf cavity where most melting occurs. According to the T–S diagrams, the winter water masses at mid-depth in the TIS cavity ( Supplementary Fig. S2 ), where most melting occurs, are found near the densest end member on the cavity mixing curve (blue points in Fig. 4 ) for both the 2001 and 2009 simulations. The densest water of year 2009, however, is warmer and more saline than that of 2001. In both simulations, the densest cavity water is situated between the densest end members of the mCDW and the polynya water mixing curves. Yet, while the denser part of the mCDW curve shows little change between the two simulations, the 2001 polynya mixing curve is much cooler and more homogenous with the appearance of more saline water near the freezing point as an end member of the curve (Low Salinity Shelf Water (LSSW), Fig. 4 ). The mixing curve of the cavity water shifts in tandem with that of the polynya, indicating more mixing at the densest end with the cold water originating in the polynya. We propose that this enhanced advection of cold polynya water into the TIS cavity is the main factor in lowering the melting rates of year 2001 simulation. To further demonstrate this connection we conduct passive tracer experiments. Tracers are initialized at the surface in the polynya areas ( Supplementary Fig. S3 ) to a value of 1 and restored to this value every hour. These passive tracers do not affect the density of the water, and therefore do not interfere with the physics of the ocean. During sea ice formation in the polynya, the tracers convect to deeper layers where they join with the coastal current and are then advected into the sub-ice-shelf cavities. Indeed, despite being released on January 1, water from the polynya begins to enter the cavities in significant quantities only in June or later ( Fig. 5 ). This attests to the role of air-sea buoyancy loss, sea ice formation and brine rejection in destabilizing water column stratification and driving convection. Before sea ice formation, the passive tracers remain in the top layers of the water column and advect westwards with the main circulation out of the model’s western open boundary. Figure 5 illustrates the large difference between the two simulations in the volume of polynya water flowing into the TIS cavity and how long it persists. 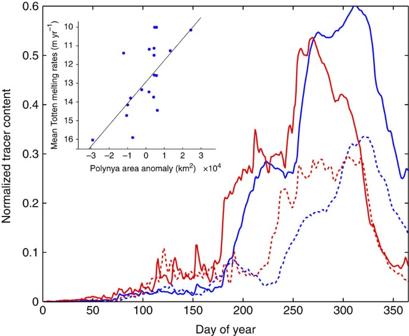Figure 5: Modelled passive tracer concentrations in the Totten and Moscow University sub-ice-shelf cavities. The passive tracers are released continuously starting on January 1 at the surface of the polynya areas nearest to TIS (blue) and MUIS (red) ice shelves and tracked during the simulation years 2001 (solid lines) and 2009 (dashed lines). Theyaxis represents the portion of cavity volume cells having tracer concentration of >0. The inset shows the correlations between mean polynya area anomalies in June–July of each simulation year 1992–2011 and the mean TIS melting rates in the following September–October of the same year. The linear correlation coefficient=0.60 and the correlation probability=0.49%. While in 2009 polynya waters begin to increase in the cavity at around day 240, reaching a maximum of ~30% of the volume cells, in year 2001 the cavity starts filling at around day 180, after which it increases rapidly to reach more than 60% of the volume cells. Furthermore, the difference between the two simulation years is more pronounced in the case of TIS than in that of MUIS. So while the area under the curve in Fig. 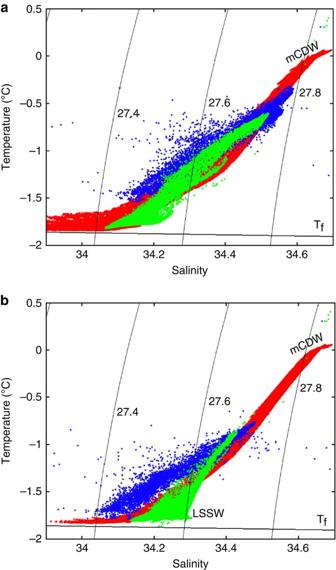5 for the 2009 simulation of MUIS is ~59% of that of the 2001 simulation, the corresponding number in the case of TIS is ~46.5%. Figure 4: The mean T-S diagrams for the August 2001 and 2009 simulations. T-S diagrams show the mixing curves for water in the Totten sub-ice-shelf cavity (blue), the polynya area (green) and an area on the continental shelf (red) in 2009 (a) and 2001 (b). The three areas are outlined by black boxes inSupplementary Fig. S1. The solid grey lines are contours of constant potential density anomaly lines. The solid black line represents the surface freezing point temperature Tf. LSSW, Low Salinity Shelf Water; mCDW, modified Circumpolar Deep Water. Figure 4: The mean T-S diagrams for the August 2001 and 2009 simulations. T-S diagrams show the mixing curves for water in the Totten sub-ice-shelf cavity (blue), the polynya area (green) and an area on the continental shelf (red) in 2009 ( a ) and 2001 ( b ). The three areas are outlined by black boxes in Supplementary Fig. S1 . The solid grey lines are contours of constant potential density anomaly lines. The solid black line represents the surface freezing point temperature T f . LSSW, Low Salinity Shelf Water; mCDW, modified Circumpolar Deep Water. Full size image Figure 5: Modelled passive tracer concentrations in the Totten and Moscow University sub-ice-shelf cavities. The passive tracers are released continuously starting on January 1 at the surface of the polynya areas nearest to TIS (blue) and MUIS (red) ice shelves and tracked during the simulation years 2001 (solid lines) and 2009 (dashed lines). The y axis represents the portion of cavity volume cells having tracer concentration of >0. The inset shows the correlations between mean polynya area anomalies in June–July of each simulation year 1992–2011 and the mean TIS melting rates in the following September–October of the same year. The linear correlation coefficient=0.60 and the correlation probability=0.49%. Full size image The T–S diagrams ( Fig. 4 ) combined with the passive tracer experiments ( Fig. 5 ) and the temperature sections in the sub-ice-shelf cavity ( Supplementary Fig. S2 ) leave little doubt that the enhanced influx of colder polynya waters into the cavity lowers the temperature and consequently reduces the simulated melting rates. This connection is further emphasized by the strength of the correlation between polynya area changes and TIS melting rates (inset of Fig. 5 ). Like TIS, tracer concentrations in the MUIS cavity are higher in the year 2001, but the difference between the two years is noticeably less ( Fig. 5 ). This is a manifestation of the more restricted connection between the MUIS sub-ice-shelf cavity and the circulation on continental shelf, which may be contributing to its lower melting rate variability ( Fig. 2 ). The better connection of TIS is possibly due to its longer ice-shelf front and the wider entrance opening along this front. Furthermore, the bathymetry in front of TIS ( Supplementary Fig. S1 ) supports the formation of an anticyclonic gyre that transports warm water to the TIS cavity entrance. These factors make the TIS cavity more susceptible to changes in conditions on the continental shelf. Hence, TIS’s higher heat influx produces higher simulated melting rates over larger areas compared with MUIS ( Fig. 3 ), but also its higher cold polynya water influx during winter leads to more effective suppression of melting. Implications for the observed Totten ice-shelf thinning In the preceding sections, numerical sensitivity simulations demonstrated the susceptibility of ice-shelf basal melting rates to changes in the volume of polynya water that reaches the cavity. Guided by this modelling insight, we propose that the observed increased thinning of the TG could be the result of sustained reduction in the volume of cold polynya water in the TIS cavity leading to higher melting. Available observations agree with certain aspects of this hypothesis. Oceanographic field measurements in the Sabrina Coast area revealed intrusions of the warm and saline mCDW occupying the deepest part of the water column [20] , [21] . This led to the suggestion that this dense water mass is a persistent feature on the shelf and capable of reaching the grounding line of TIS [20] . Our modelling results support the contribution of mCDW to the water mass in the sub-ice-shelf cavity. Observed glacier thinning has been attributed to a possibly enhanced onshore flow of warm mCDW into the cavity [20] . Here we propose another mechanism based on the reduced flow of cold polynya water. We examined the occurrence of polynyas in the vicinity of the two ice shelves by analysing the Kern data set [22] , [23] of daily polynya/thin ice locations (see Methods). 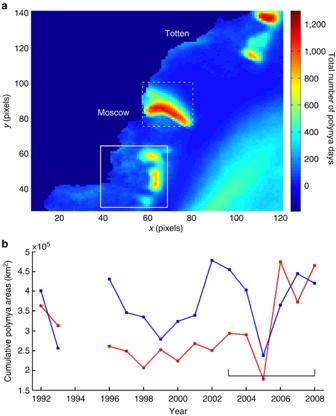Figure 6: Polynya observations in the vicinity of Totten and Moscow University ice shelves. Data were obtained from the Kern PSSM set22,23. The years 1994 and 1995 were not included in either panel because of missing data. (a) Total number of polynya days occurring at each pixel location on the continental shelf off of the two ice shelves (domain is similar toSupplementary Fig. S1) for the months June to September during the years 1992–2008. Pixels are 5 × 5 km. (b) Time series of the cumulative area of polynyas occurring in the months June to September of each year nearest to TIS (blue) and MUIS (red). The series for Totten was calculated for the area in the dashed rectangle in (a) and in the rectangle for Moscow. The black square bracket indicates the ICESat-1 observation period. Figure 6a shows the Dalton coastal polynya that is located east of the TIS front roughly between longitudes 120 and 121 °E, and the polynya that forms east of MUIS between 123 and 124 °E, as was observed in previous studies [24] , [25] . The areal extent of latent heat polynyas can be used as a proxy for sea ice production levels [25] , [26] , and hence for the rates of ocean heat loss and salinity increase due to the process. We obtained a time series of the areal extents of the polynyas nearest to TIS and MUIS (see Methods) for the period 1992–2008. The results ( Fig. 6b ) do not reveal a discernible secular trend. They do show however that the areal extent of the TIS polynya was increasing from 1999 to 2002, after which it declined to notably lower levels in 2004, 2005 and 2006. It recovered thereafter but remained below or at the 2002 and 2003 levels. The drop in polynya extent in the middle part of the ICESat-1 observation period (2003–2008; Fig. 6b ) relative to its 2003 level must have reduced the amount of sea ice production and the accompanying formation of cold and saline water. This finding lends further support to our hypothesis that the decrease in the volume of cooler water mass reaching the sub-ice-shelf cavity would have contributed to increased TIS melting rates and the observed cumulative thinning. Support also comes from the observed increase in the areal extent of the polynya east of MUIS in the years of the ICESat-1 period, except for 2005, consistent with the small surface elevation change observed in the MUG area. Figure 6: Polynya observations in the vicinity of Totten and Moscow University ice shelves. Data were obtained from the Kern PSSM set [22] , [23] . The years 1994 and 1995 were not included in either panel because of missing data. ( a ) Total number of polynya days occurring at each pixel location on the continental shelf off of the two ice shelves (domain is similar to Supplementary Fig. S1 ) for the months June to September during the years 1992–2008. Pixels are 5 × 5 km. ( b ) Time series of the cumulative area of polynyas occurring in the months June to September of each year nearest to TIS (blue) and MUIS (red). The series for Totten was calculated for the area in the dashed rectangle in ( a ) and in the rectangle for Moscow. The black square bracket indicates the ICESat-1 observation period. Full size image To test whether the thinning of TG did actually increase during the ICESat-1 period, we examine in detail surface elevation change patterns along three sections ( Fig. 1a ) in the part of the glacier with the most observed surface lowering. The profiles in Fig. 1b show that most surface lowering occurred in the latter part of the period (the blue points). In fact, when considering the slower-flowing areas at the flanks of the glacier (north of −67.2° and south of −67.8°) all of the surface lowering appears to have occurred in the latter part of the period as all four profiles are overlapping. This spatial difference also suggests that while the faster-flowing areas have been lowering throughout the ICESat-1 period, the slower-flowing flanks started thinning only later during the period. This lag in the onset of thinning at the flanks suggests that the perturbation causing it must have been recent. Supplementary Fig. S4a shows similar patterns further upstream. The profile with the longest time span (blue) depicts the most surface lowering as expected. The other two profiles cover shorter periods, with the one occurring later in the period (cyan) showing more surface lowering than the one occurring earlier (green). Again, all three profiles overlap on the flank (north of −67.2°). In Supplementary Fig. S4b , the profiles are more noisy as the surface elevation change signal is smaller this far upstream, but it can still be discerned that in the section between −67.8° and −68.3° the profile occurring later (blue) shows more surface lowering than the one occurring earlier (green). These analyses of surface elevations changes indicate that the thinning of TG did indeed increase during the ICESat-1 observation period. This, combined with the findings of reduced polynya extents in the same period, provides persuasive observational evidence in support of our hypothesis. To summarize: while the TIS polynya extent ended the 2003–2008 period close to its level at the start, throughout that period it was less than the 2003 extent, markedly so for some years, and each such reduced polynya episode would have been associated with enhanced TIS melting. The enhanced melting during each episode would contribute to the cumulative signal of thinning measured over the observation period. The occurrence of the most reduced polynyas between 2004 and 2006 is consistent with the cumulative thinning of TIS being observed to have increased in the latter part of the 2003–2008 observation period. The case for closer study of the region encompassing Totten and Moscow University glaciers and ice shelves is accentuated by its large ice volume discharge into the ocean, the rapidity of the observed changes and the recently discovered complexity of the basal topography beneath the drainage basin of the two glaciers [12] . That large parts of the basin lie beneath sea level, with the deepest regions hundreds of kilometres inland [11] , [12] , raises the question of whether TG could become the Pine Island of East Antarctica. This study explored possible underlying processes. The numerical simulations demonstrated the role of cold polynya water in modulating melting rates in the sub-ice-shelf cavity, as well as provided support for the idea of the persistence of mCDW on the continental shelf and its suggested reach into the cavity [20] . Based on these modelling insights, we proposed that the observed increased thinning of TG could be a consequence of the sustained reduction in the volume of cold polynya water reaching the sub-ice-shelf cavity. This hypothesized connection has wider implications. The colder and more saline water mass resulting from sea ice formation has hitherto mostly been studied in the Weddell Sea sector of Antarctica [27] , where it is referred to as High Salinity Shelf Water (HSSW). While in that context HSSW is the agent of sub-ice-shelf melting, our findings suggest that in other circumstances the water resulting from sea ice production can have the opposite effect of subduing melting at the ice–ocean interface. These differing roles of the polynya water are largely due to the dominance of HSSW in the southern Weddell Sea even during summer [27] , favored by a broad continental shelf and the presence of land to the west [28] , contrasted with the intrusion of the warm and saline mCDW [20] on the much narrower continental shelf off of Totten and Moscow University ice shelves. We therefore explain increased melting in the sub-ice-shelf cavity not by an encroachment of CDW or an increase in the temperature of existing water masses as is usually suggested, but rather as a consequence of the reduction or absence of a certain cooler water mass. This process is generally overlooked, yet our findings strongly call for it to be considered in other locations, especially in view of the well-documented changes in sea ice conditions around Antarctica and Greenland. Candidate locations combine a number of criteria. They are mainly glaciers that flow into ocean basins having narrow continental shelves that allow encroachments of warm CDW to reach the sub-ice-shelf cavities, but also having relatively strong Antarctic Slope Fronts that would prevent CDW from overwhelming the cavities, hence allowing locally produced cold water masses (such as in polynyas) to affect sub-ice-shelf cavity processes. Variability in CDW may well be contributing to the observed TG thinning, but the paucity of in situ hydrographic data did not allow effective examination of this possibility. In a future pursuit of the investigation here, this and other questions would benefit greatly from better knowledge of the ocean hydrographic variability, as well as from more accurate continental shelf bathymetry and cavity geometry such as being generated by Operation IceBridge elsewhere in Antarctica. Finally, previous studies of Wilkins [8] and George VI [29] ice shelves proposed that these ice shelves were affected by changes in local conditions on the continental shelf. Unlike most Antarctic ice shelves, however, George VI and Wilkins are characterized by shallow drafts that lie mostly in the top layers of the water column putting them directly in contact with hydrographic conditions there. The findings here, on the other hand, demonstrate that melting rates in the deep cavities beneath thick ice shelves that drain large basins can be sensitive to hydrographic changes on the adjacent continental shelf. In this study, we investigated hydrographic changes due to latent heat polynya variability. Many local factors combine to determine where a polynya forms and how large and persistent it is, including ice-sheet topography, shoreline geometry, ocean bathymetry, grounded icebergs and winds [24] , [28] . Hence, from the exploration here of interactions among ice shelves, ocean, sea ice and atmosphere emerges the key role of processes occurring on a smaller geographic scale in determining the specific manner in which large-scale climatic variability may translate into ice-shelf instability. GLAS/ICESat-1 data and firn compaction model We calculate surface elevation differences from the measurements of the Geoscience Laser Altimeter System (GLAS) that was carried on the Ice, Cloud and land Elevation Satellite (ICESat-1 (ref. 30 )), using the GLA12 product (Level 2 Antarctic and Greenland Ice Sheet Altimetry Data) of Release 633, the most recently available [31] . GLAS/ICESat operated during the period 2003–2009, making measurements two or three times a year during ‘campaigns’ lasting 4–5 weeks in most cases (we did not find useable data from the 2009 campaigns). Surface elevation changes are calculated by an along-track method [2] , [32] . Our implementation of this method consists of taking two parallel ICESat-1 tacks from the same year or from two consecutive years, to which we refer as the base tracks. We create a plane Delaunay triangulation of the set of points lying on the two tracks. Only triangles with circumcircles having radii ≤200 m are included in the analysis. The triangulation then forms the basis for computing a field of linearly interpolated surface elevations. To find surface elevation differences relative to a track from a later or an earlier year, points of that track that lie between the two base tracks are first identified. The difference is then calculated between the elevation of each identified point and the elevation at its corresponding location in the interpolated field. We refer to each group of three tracks used for such surface elevation change calculation as a track combination. The combinations are listed in Supplementary Table S1 . The effects of firn layer depth variability on elevation are calculated by a firn densification model [33] . The model simulates the evolution of firn depth at a sub-daily temporal resolution and a horizontal spatial resolution of 27 km. Surface mass balance, snow melting and meltwater percolation and refreezing are represented, and the model is forced at the surface by the Regional Atmospheric Climate Model (RACMO2) [46] . Data are filtered and corrected for tidal and atmospheric effects before calculating elevation differences. Thus, data points flagged as invalid are removed, as well as points having saturation correction flag (parameter i_satCorrFlg) values >2. The remaining points are adjusted with the appropriate saturation elevation correction (parameter i_satElevCorr). Measurements that might have been affected by clouds are filtered out with the detector gain (parameter i_gval_rcv), only allowing measurements with gain ≤80 counts [34] , [35] , [36] . Load tides are applied with the TPXO6.2_load medium-resolution, global inverse model [37] . Further corrections are needed for points on the floating ice shelves due to tides and changes in atmospheric pressure. The effect of ocean tides is calculated with the high-resolution (4 km) CATS2008a_opt regional model of the circum-Antarctic ocean [38] , which assimilates available remote sensing and in situ tidal observations. The isostatic response of the ice shelf to changes in atmospheric pressure, known as the inverse barometer effect [39] , is calculated using the value of 1.12 cm of surface elevation lowering for each 1 millibar of increase in atmospheric pressure [35] . The uncertainty of GLAS/ICESat-1 elevation measurements on grounded ice is assessed to be 14 cm (ref. 40 ). Uncertainty associated with the model correction for load tide is estimated to be ~0.5 cm (ref. 41 ). A maximum uncertainty in firn layer surface elevation values of ~9 cm is calculated for the study area [33] (see also ref. 3 ). Assuming that these uncertainties are random and independent, the combined uncertainty is ~16.7 cm on grounded ice. On floating ice, the CATS2008a_opt tide model adds a further uncertainty of 7.8 cm (ref. 42 ) and the barometric correction another ~2 cm, based on ~2 millibar error in surface atmospheric pressure [43] . The combined uncertainty of ice-shelf surface elevations is therefore ~18.5 cm. When calculating the change in surface elevations, propagation of error produces uncertainties that are twice those of the individual measurements of surface elevation, as noted in Fig. 1b and Supplementary Fig. S4 . Average melting rates from remote sensing observations We estimate the area-averaged ice-shelf melting rates using remote-sensing data by applying mass conservation between a flux gate at the glacier grounding line and another gate near the ice-shelf front. Mass flux is calculated as the product of thickness and velocity integrated across each flux gate. Ice thickness at the grounding line from NASA Operation IceBridge [44] , and thickness at the near-front gate [10] , are used with ice velocity at both gates from MEaSUREs [45] . We obtain the surface mass balance for the area between the grounding line and the front gate of the ice shelf from the simulations of RACMO2 (ref. 46 ). Assuming steady state conditions, the inferred basal melting rates of TIS and MUIS are listed in Table 1 . Ice–ocean interaction model We simulate ice–ocean interaction with the Massachusetts Institute of Technology general circulation model (MITgcm), which includes a dynamic/thermodynamic sea-ice model [47] . Freezing/melting processes in the sub-ice-shelf cavity are represented by the three-equation-thermodynamics [48] with modifications [49] as implemented in MITgcm [50] . Exchanges of heat and freshwater at the base of the ice shelf are parameterized as diffusive fluxes of temperature and salinity using the constant turbulent exchange coefficients [51] . Initial conditions and boundary conditions for hydrography and sea ice are provided by a coarse resolution (18-km grid) Estimating the Circulation and Climate of the Ocean Phase II (ECCO2) adjoint solution [52] . The model domain ( Supplementary Fig. S1 ) is derived from the global configuration used by ECCO2, but with horizontal grid spacing of ~1 km and a vertical discretization of 70 vertical levels of varying thickness (10 m at the surface to 450 m at the deepest level). Bathymetry is based on the Smith and Sandwell topography version 14.1 (ref. 53 ), ice-shelf thicknesses are from the Griggs and Bamber data [10] and grounding line positions are from Rignot et al. [54] With these data, the sub-ice-shelf cavity bathymetries are approximated with varying water column thickness by adding to the observed ice-shelf thickness a linearly increasing gap ranging from 35 m at the grounding line to 250 m at the mouth. In these cavities, grid cell vertical dimensions are maintained at <30 m to enhance the modelling accuracy. On the other hand, the relatively high vertical resolution combined with the 70 vertical-level model discretization constrain simulations in the sub-ice-shelf cavities to a maximum depth of 1,750 m ( Supplementary Fig. S2 ). However, the narrowness of the cavity below this depth ( Supplementary Fig. S2 ) means that what is being excluded from the cavity volume is a relatively small portion that is most vulnerable to spurious simulated melting rates due to its limited exchanges with the rest of the cavity. The original bathymetry product contains a shallow ridge in front of the ice shelves—an unobserved artifact arising from the interpolation of sparse bathymetry data from the shelf to the shoreline. The artificial ridge prevents the exchange of water masses between the sub-ice-shelf cavities and the continental shelf. To allow the exchange of water between the shelf and the sub-ice-shelf cavity, we remove the artificial ridge in the immediate vicinity of the cavities. Owing to the difference in resolution between the 18-km model and the 1-km model domain, a relaxation (20 grid points into the model domain) is applied to temperature and salinity along the open boundaries to avoid artifacts such as wave energy radiating into the model interior. Surface atmospheric forcing is derived from the Japan Meteorological Agency and Central Research Institute of Electric Power Industry 25-year reanalysis (JRA-25 (ref. 55 )). A best fit of the simulated sea ice concentrations to the available observational data is found by adjusting sea-ice model parameters in ECCO2, forced with JRA-25, using the Green’s function approach [56] . We have successfully applied a similar configuration of this model in a study of Pine Island Ice Shelf [57] . Here we conduct 20 model experiments for the years 1992–2011. Each experiment consists of a 1-year model integration with identical initial and lateral ocean boundary conditions derived from an ECCO2 global adjoint solution, while allowing the surface forcing fields from JRA-25 to vary from year to year. Polynya extents We analyse polynya presence using the Kern data set [22] , which is derived for the years 1992–2008 from measurements made by the Special Sensor Microwave/Imager (SSM/I) using the Polynya Signature Simulation Method (PSSM) [23] . Polynyas are defined as areas in the sea ice cover that are either open water or <20 cm thick. Mean daily winter polynya areas are provided at a spatial resolution of 5 km and an uncertainty estimated to be 80–250 km 2 (ref. 23 ). We find the time series of polynya extents in the two areas outlined in Fig. 6a over the coverage period, excluding the years 1994 and 1995 because of their data gaps. We devise a simple parameter that represents both the areal extent of polynyas and how long they lasted for each year. Hence, for every June, July, August and September day of each year in the time series, the counts of pixels identified as polynya are added to form the cumulative value for that year, which is then expressed in km 2 . How to cite this article: Khazendar, A. et al. Observed thinning of Totten Glacier is linked to coastal polynya variability. Nat. Commun. 4:2857 doi: 10.1038/ncomms3857 (2013).